Coherent diffraction imaging of nanoscale strain evolution in a single crystal under high pressure The evolution of morphology and internal strain under high pressure fundamentally alters the physical property, structural stability, phase transition and deformation mechanism of materials. Until now, only averaged strain distributions have been studied. Bragg coherent X-ray diffraction imaging is highly sensitive to the internal strain distribution of individual crystals but requires coherent illumination, which can be compromised by the complex high-pressure sample environment. Here we report the successful de-convolution of these effects with the recently developed mutual coherent function method to reveal the three-dimensional strain distribution inside a 400 nm gold single crystal during compression within a diamond-anvil cell. The three-dimensional morphology and evolution of the strain under pressures up to 6.4 GPa were obtained with better than 30 nm spatial resolution. In addition to providing a new approach for high-pressure nanotechnology and rheology studies, we draw fundamental conclusions about the origin of the anomalous compressibility of nanocrystals. Pressure drastically changes material properties and reveals surprising physical [1] , [2] and chemical [3] phenomena, novel materials [4] and the nature of deep Earth and planetary interiors [5] , [6] . Extreme pressures are reached at diminishingly small sample volume. Recent progress in high-pressure science is dictated by the capability in probing microscopic samples in situ in diamond-anvil cells (DACs) [7] . The high-pressure environment prohibits the use of vacuum-based nanoscale technology, such as electron microscopy, nanoSIMS, atomic force microscopy and so on. High-energy X-ray is the only source capable of nanoscale resolution that can penetrate through the diamond anvils or the surrounding materials, but has been previously limited to diffraction studies of bulk or aggregate properties [8] or imaging of 100-μm sized samples with μm resolution [9] . The recent developed depth-resolved X-ray diffraction technique can provide internal strain distribution along the beam penetration direction with about 1 μm point-to-point spatial resolution, providing crystal orientation and strain information for mesoscale structural analysis [10] . To study nanometre-sized grains, a much higher spatial resolution probe is required. The Bragg coherent X-ray diffraction imaging (CXDI) technique is a promising tool to probe the internal strain distribution of individual nanometre-sized single crystals [11] . Coherence is a property that can be imposed on an X-ray beam by setting an entrance slit smaller than the transverse coherence length. X-ray beams generated by third-generation sources of synchrotron radiation using undulators have practical levels of flux after the pinhole small enough to ensure coherence in the range of 10 9 photon s −1 . As the coherent X-rays pass through a distorted crystal, both the scattering intensity and phase will be affected. Bragg CXDI operates by inverting three-dimensional (3D) diffraction patterns in the vicinity of Bragg peaks to real-space images using phase retrieval algorithms [12] . In the resulting images, the reconstructed magnitude represents the electron density of the crystal, while the obtained phases are attributed to lattice distortions projected onto the Bragg direction. CXDI is also called lens-less microscopy, as the diffracted wavefield Fourier components are transferred back in real space numerically without a microscope. Typical CXDI beamline uses the least optical components possible in the beam path from source to detector to preserve the transverse coherence. So long as the beam is also sufficiently monochromatic, it will then have full spatial coherence [13] . In the case of partially coherent illumination, the recorded intensity is given by [14] , [15] , [16] where γ ( x ) and ( q ) are the so-called mutual coherence function (MCF) and its Fourier transform, and x is the separation in the plane of the sample. The scalar wavefield ψ ( x ) and scalar diffracted wavefield ^ ψ ( q ) are complex. Unlike the direct phase retrieval method used for ideal full coherent diffraction case, both the wavefield and MCF are updated at each step of the iterative phase retrieval calculation until both quantities converge. This method has been successfully demonstrated for Au nanocrystals similar to those used in this work [15] . The de-convolution of the MCF turned out to be crucial to the full coherent imaging of our studies presented here. For in-situ static high-pressure study, DAC is the most common apparatus to generate pressure up to multi-megabar. The sample is inserted between two anvils made of diamond inside the hole of a gasket and surrounded by a pressure-transmitting medium. X-rays need to pass through either the diamond anvils or the gasket and the pressure medium. Although the single crystal diamond anvils should have less distortion than the beryllium gasket under pressure, more than 80% of X-ray intensity will be absorbed by two anvils for the energy we used for CXDI (10.8 keV) and forward direction has limit angular opening for reciprocal space. We decided to let X-rays pass through the beryllium gasket, which can significantly affect the wavefront of the beam. Especially when these components are refractive, this could have a deleterious impact on the ability to obtain an image by CXDI, because it restructures both the beams entering and leaving the sample environment. Strictly, the degree of coherence of the beam, described by MCF is determined by the undulator synchrotron radiation source alone and should not be affected by this inadvertent optical distortion [14] . However, if the optical distortion is not too strong, its effect can be folded in with the pre-existing MCF of the source to make an effective MCF with smaller coherence lengths. This is achieved by averaging diffraction patterns of the same crystal with slightly different alignments, such as position on the beam and small rotations about the q-vector. We can then use the method of Clark et al . [15] to de-convolute the observed diffraction patterns and obtain both the 3D morphology and phase distribution of the studied crystal. As the effective MCF is modified by the changes of the sample that surround the environments (pressure medium density, beryllium gasket thickness and so on with pressures), the effective MCF was obtained by modelling to optimize the output. Strain sensitivity better than 1 × 10 −4 and spatial resolution better than 30 nm can be achieved. The mechanical properties of nanoscale gold particles have attracted considerable interest for tailoring the properties of molecular electrodes, nanoscale coatings and advanced engineering materials [17] , [18] , [19] . A recent high-pressure powder diffraction study on 30 nm gold particles [20] has shown they have 60% higher stiffness compared with micron-size counterparts. Our CXDI method can provide detail 3D morphology and strain distribution within single nanocrystal at a few tens of nanometre spatial resolution, which is crucial to understand the micromechanism of the enhanced stiffness. Hence exploring the mechanical response of gold crystals under high pressure at nanometre scale can impact both fundamental physics and applied sciences. When a gold crystal is under a quasi-hydrostatic pressure in a DAC, any shear stress will create a boundary condition to affect the internal strain distribution, which could create lattice distortions, morphology change and plastic flow as the applied external pressure increases. Here we report the Bragg CXDI studies on the strain and morphology evolution of a single 400-nm sized gold crystal with 30 nm resolution as the pressure change to gain insight on the possible nanoscale mechanism of its high-pressure response. Reconstruction procedure with MCF The schematic of the experimental setup is shown in Fig. 1 . 3D diffraction patterns from the same gold crystal in a DAC were collected at several pressure conditions up to 6.4 GPa (see Methods section). To reduce the systematic effects of wavefront distortion, typically 5–8 repeated scans were collected at each pressure point, under slightly different alignment conditions, and averaged together. The diffraction data were inverted using phase retrieval algorithms, which utilize sufficiently oversampled diffraction intensities to recover the unmeasured phases of diffraction signal. In the reconstruction process, known information is imposed as constraints. The usual constraints are modulus constraint, which requires that the calculated Fourier intensity agrees with the measured data, and support constraint, which assumes that the sample is finite and isolated from other scatters in real space. We used a reconstruction cycle with an algorithm sequence of 10 error reduction, 150 hybrid-input-output and 40 error reduction. The ‘shrink-wrap’ strategy was used to refine the crystal shape used as a support [21] . 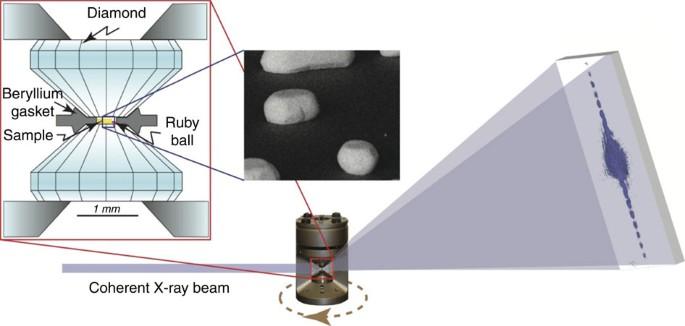Figure 1: Overall schematic of the experimental setup. A large opening panoramic diamond-anvil cell is used to compress the studied crystal, positioned at the rotation centre of the diffractometer. An X-ray sensitive charge-coupled device is placed at 1 m away to collect far-field diffraction patterns. The insert scanning-electron microscopy (SEM) picture shows typical gold nanoparticles distributed on a silicon substrate. The zoomed-in figure of the DAC shows the sample environment. Figure 1: Overall schematic of the experimental setup. A large opening panoramic diamond-anvil cell is used to compress the studied crystal, positioned at the rotation centre of the diffractometer. An X-ray sensitive charge-coupled device is placed at 1 m away to collect far-field diffraction patterns. The insert scanning-electron microscopy (SEM) picture shows typical gold nanoparticles distributed on a silicon substrate. The zoomed-in figure of the DAC shows the sample environment. Full size image To de-convolute the influence of beam disturbance by the DAC gasket and pressure medium, modelled as a modified MCF, we used the method developed for CXDI with partial coherence [15] . The MCF is convolved with the calculated Fourier modulus before applying the modulus constraint. The unknown MCF function is updated regularly using iterative Richardson-Lucy algorithm [22] , [23] . The searching criterion is to minimize the difference between the measured data and the convolution of this characterization function with calculated Fourier modulus. The reconstructed images using data measured at the initial pressure 0.8 GPa with and without partial coherence correction are shown in Fig. 2a . We found that the coherence correction gives a smoother crystal boundary and significantly improves the algorithm’s convergence, as found previously by Clark et al . [15] The corresponding MCF function for this data set is plotted in Fig. 2b . The extracted MCF is a 3D function that includes the transverse coherence properties in the XY-plane, perpendicular to the incident X-ray beam direction, and the temporal (or longitudinal) coherence properties related to the monochromaticity of the wavefield along its Z-direction. The effect of applying the MCF is to blur the coherent intensity from measured sample by convolving it with the Fourier transform of the MCF [14] , [15] . The comparison of the original measured and de-convoluted diffraction intensity distribution at 0.8 GPa is shown in Supplementary Fig. S1 . The MCF, along X, Y and Z directions, is plotted in Fig. 2b , from where one can see from the smooth decay of the MCF that any pair of points separated by some distance are partially coherent. 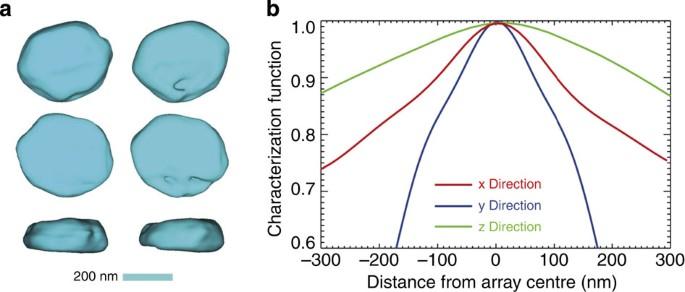Figure 2: Impact of the mutual coherence function (MCF) on the reconstructed images at 0.8 GPa pressure. The reconstructed amplitude plots at top, bottom and side views with (left) and without (right) MCF correction (a), and the corresponding line profiles along x and y (lateral), and z (longitudinal) directions of the MCF (b). The characterization function is a three-dimensional description of the degree of coherence between any two points with a certain distance along x, y, and z directions from an array centre. Figure 2: Impact of the mutual coherence function (MCF) on the reconstructed images at 0.8 GPa pressure. The reconstructed amplitude plots at top, bottom and side views with (left) and without (right) MCF correction ( a ), and the corresponding line profiles along x and y (lateral), and z (longitudinal) directions of the MCF ( b ). The characterization function is a three-dimensional description of the degree of coherence between any two points with a certain distance along x, y, and z directions from an array centre. Full size image 3D reconstructions of morphology and phase under pressures As seen in the scanning-electron microscopy image of the gold nanoparticles in Fig. 1 , the individual particles often adopt a faceted morphology, probably related to the equilibrium crystal shape at the annealing temperature. 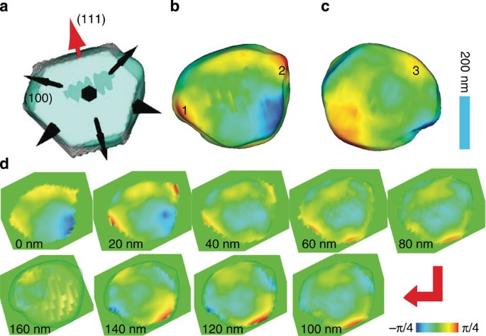Figure 3: 3D morphology and strain distribution of the gold crystal at 1.7 GPa. (a) Isosurface (30%) of the reconstructed amplitude superimposed with a model of the possible {111} and {100} crystal planes. The normal directions of two sets of crystalline planes {111} and {100} are marked by two kinds of arrows (fat and narrow), and the one (111) used for the measurement is marked in red. (b,c) are the top and bottom view of phase shift distribution pasted on the 30% isosurface plot. Three strain distinguished locations numerically labelled are chosen for quantitative measurement as a function of pressure. (d) 3D phase distribution at different slicing depths spaced apart by 20 nm steps from top to bottom of the crystal. The colour scale is used to show the relative phase shift and normalized to range [−π/4, π/4]. Figure 3 displays the reconstructed results of the 400 nm crystal at 1.7 GPa. The magnitude of the reconstructed density ψ ( x ) at its 30% isosurface is shown in Fig. 3a . The surface normal is along (111) direction and the crystal shape shows a good threefold symmetry. We notice that all surface facets can be described as either {111} or {100} crystalline planes, as it is known that the {111} and {100} facets are the most stable planes for Au. A tight wrap model, defined by all {111} and {100} planes, is overlaid with the 30% isosurface object in Fig. 3a . Fat and narrow arrows denote the {111} and {100} plane normal directions, respectively. The arrow labelled as red in Fig. 3a represents the q-vector direction of the Bragg reflection used. Figure 3b are the top and bottom view of phase shift, respectively. The colour shows the phase shift relative to the average phase of entire particle, set to zero. The phase shift colour is normalized to range [−π/4, π/4]. The bottom two rows in Fig. 3 are slices through the 3D reconstructed phase object in 20 nm depth steps running from the top to bottom. One can see the high-strain areas are mainly located at the corners where two {111} planes and one {100} plane intersect. The interior volume is nearly strain free. Three distinguished corners marked as 1, 2 and 3 in Fig. 3b were selected for further quantitative strain analysis as applied pressure increases. Figure 3: 3D morphology and strain distribution of the gold crystal at 1.7 GPa. ( a ) Isosurface (30%) of the reconstructed amplitude superimposed with a model of the possible {111} and {100} crystal planes. The normal directions of two sets of crystalline planes {111} and {100} are marked by two kinds of arrows (fat and narrow), and the one (111) used for the measurement is marked in red. ( b , c ) are the top and bottom view of phase shift distribution pasted on the 30% isosurface plot. Three strain distinguished locations numerically labelled are chosen for quantitative measurement as a function of pressure. ( d ) 3D phase distribution at different slicing depths spaced apart by 20 nm steps from top to bottom of the crystal. The colour scale is used to show the relative phase shift and normalized to range [−π/4, π/4]. Full size image The Bragg CXDI measurements were performed at 0.8, 1.7, 2.5, 3.2 and 6.4 GPa on the same crystal. The reconstructed images (both top and bottom views) are shown in Fig. 4a . The dimension of the measured crystal is about 480 × 380 × 180 nm at 0.8 GPa and shrinks a little bit as pressure increases. The noteworthy features in Fig. 4 are the morphology change and strain redistribution as pressure increases. The phase shifts as a function of pressure at the selected three distinguished locations are plotted in Fig. 4b . At each selected corner region, the phase shift values within 3 × 3 × 3 pixel boxes with pixel size 12 nm around the centre were taken, and the averaged values were plotted as a function of pressure in Fig. 4b , where the maximum and minimum values in the 3 × 3 × 3 boxes were used as the error bar range, respectively. The phase shift value is directly connected to the local lattice displacement, thus strain, projected to the measured direction as φ = ·Δ ( [11] ). 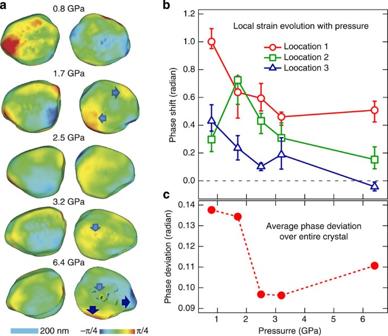Figure 4: Phase distribution as a function of applied pressure (0.8–6.4 GPa). Two-dimensional views from the top and bottom are shown ina. The quantitative phase shift values at locations 1–3 labelled inFig. 3and the deviation over entire crystal are plotted inbandcas a function of pressure. Arrows inapoint to the characteristic strain-evolving regions discussed in the text. The phase shift values inbare the averaged values within 3 × 3 × 3 pixel boxes around the centres taken at the selected corner region labelled inFig. 3, while the maximum and minimum values in the 3 × 3 × 3 boxes are used as the error bar range, respectively. Figure 4: Phase distribution as a function of applied pressure (0.8–6.4 GPa). Two-dimensional views from the top and bottom are shown in a . The quantitative phase shift values at locations 1–3 labelled in Fig. 3 and the deviation over entire crystal are plotted in b and c as a function of pressure. Arrows in a point to the characteristic strain-evolving regions discussed in the text. The phase shift values in b are the averaged values within 3 × 3 × 3 pixel boxes around the centres taken at the selected corner region labelled in Fig. 3 , while the maximum and minimum values in the 3 × 3 × 3 boxes are used as the error bar range, respectively. Full size image It is clearly seen that the strain level decreases as pressure increases, while the crystal shape evolves significantly. The starting, well-faceted shape becomes smoother around the corners, which implies large plastic flow has taken place within the sample during the compression. Location 2 is anomalous: initially the strain level was relatively low at 0.8 GPa, as at 1.7 GPa the local strain was quickly built up while a geometrically sharp corner was formed. On further compression, this sharp corner became rounder while the rest of the sample and strain level were decreasing quickly. For an fcc-Au crystal under a quasi-hydrostatic pressure condition, the lattice parameter a and hence the volume of unit cell will decrease as a dilatation strain component. The phase of average values over the entire crystal < φ i > gives the measure of this component. The phase deviation of φ i at each measured voxel from < φ i > gives the local deviatoric strain measure. For checking the overall phase shift evolution as a function of pressure, we evaluated the standard deviation of phase over the entire crystal in Fig. 4c , where phase deviation is calculated as . The overall trend is the average phase deviation decreases with pressure. A phase shift of 1.0 radian (about the highest phase shift measured here) corresponds to a lattice strain of ~2 × 10 −4 at the edge of the crystal. As the measured phase shift is only the projected component along the direction, the real strain should be larger than our observation. Overall, the strain sensitivity better than 1 × 10 −4 is achievable. Besides the dramatic changes at the selected corners, the overall strain evolution at the bottom of the crystal, the interface between crystal and substrate SiO 2 layer, was also significant. At 0.8 GPa, the bottom surface is nearly strain-free indicating the high temperature treatment when sample was formed (see Methods section) and has released the interface strain between gold crystal and SiO 2 surface well. As pressure increased to 1.7 GPa, strain started to build up at two areas away from the centre (lower-left and upper-right as indicated by two arrows). A uniform but strained distribution formed at 2.5 GPa, and a new high-strain centre reemerged near the centre (marked by arrow) of the bottom surface at 3.2 GPa. At the highest pressure measured in this work (6.4 GPa), the strain was largely relieved near the newly formed hole in the central part, but large strain has shifted to the side (bottom and right), which counts for the increasing average phase variation in Fig. 4c . A new sharp corner has emerged at the right side too. The missing part of electron density from the amplitude reconstruction implies the bottom of the crystal may have partially de-bonded from the substrate, which may be caused by high strain accumulation or X-ray damage. On further compression, we noticed this crystal disappeared from the detector even after both reciprocal and real-space searching, which indicated the crystal was totally de-bonded from substrate and rotated to a different orientation or moved out of the searching field. The usual result of high-pressure powder diffraction under quasi-hydrostatic conditions is that the diffraction peaks become broader at higher pressure, suggesting a larger strain variation. From this single crystal CXDI study, we found the opposite that the overall strain variation cross the entire crystal decreases with the applied pressure increases. This apparent discrepancy can be attributed to the fact that we examined an isolated grain in the current study, in the absence of interactions with adjacent grains. The capability of probing single nanocrystal in DAC will allow scientists to extend this type of research to ultra-high pressure study (multi-mega bars upto ten mega bars region). As the inhomogeneity of the materials (gasket and pressure-transmitting medium) in the beampath, they may introduce the distortion of the exited field. Hruszkewycz et al . [24] have made comparison of numerical simulation and experimental results from a gold crystal placed inside a beryllium dome, and found that a critical length scale feature (void size) L = Dλ / d obj gave the most distortion to the exited field. As our sample environment is very similar to the case Hruszkewycz et al . reported [24] , but with different dimensions, we would expect major disturbing effect from ~43 nm by 20 nm featured particles (defects, void and so on). As we measured the sample at each pressure 5–8 times with slightly different alignment condition, it is unlikely we hit this particular particle size in the beampath. The defect sizes far away from this characteristic value gave negligible effects. At different pressures, the surrounding materials around the sample change, which leads the change on effective MCFs ( Supplementary Fig. S2 ). CXDI provides unprecedented spatial resolution, but limit to sample size to view due to the limit coherent lengths. Recently developed X-ray ptychography allows to measure larger sample without suffering the spatial resolution [25] . We expect that this technique will be available to high-pressure research to expand our research to a larger-scale research. In summary, the 3D evolutions of morphology and strain distribution in ~400-nm gold crystal were measured with better than 30-nm spatial resolution and 1 × 10 −4 strain sensitivity by Bragg coherent diffraction imaging technique under an applied pressure from 0.8 GPa to 6.4 GPa in a DAC. This gives big improvements of about two orders of magnitude in 3D spatial resolution and one order of magnitude in strain determination for high-pressure study. Once de-convoluted from a MCF, the coherent diffraction patterns were successfully reconstructed and inverted to 3D images. On increasing the applied pressure, some of the initial high-strain corners in the crystal shape reduce their strain level, while other areas acquire a sharper local geometry and higher local strain. On further pressure increases, the strain at all these locations dropped and stayed at low level. The current research for the first time demonstrates the powerful high resolution of Bragg CXDI to study the morphology and internal strain evolution under high pressure, which leads to a very promising approach for in-situ nanotechnology development under high pressures. Sample preparation The gold nanocrystals were prepared by dewetting of evaporated gold films at a temperature just below melting [26] . A 20-nm-thick gold film was deposited on silicon wafer surface. It was then annealed in air in a furnace at 1,100 °C for several hours. Isolated gold crystals were formed, about 300–400 nm in diameter, 200 nm in height and about 1 μm separation, with {111} ‘fibre’ texture on a thin layer of SiO 2 . A small piece of the silicon wafer containing gold crystals was mechanically polished down to about 15 μm from the backside to fit in the gasket hole. A panoramic DAC with a pair of 300 μm culet size diamond anvils was used for the in-situ high-pressure study. A Beryllium gasket was pre-indented to 40 μm thick and a 150 μm diameter hole was drilled in the centre to host the silicon wafer and a small ruby sphere. A mixture of methanol and ethanol (4:1) was used as pressure-transmitting medium. The pressures were monitored from the Ruby fluorescence shift [27] . Experiment The Bragg CXDI experiment was performed at beamline 34-ID-C of the Advanced Photon Source (APS), Argonne National Laboratory. A coherent 10.8 keV X-ray beam was selected by a silicon (111) double-crystal monochromator, and focused to ~1.5 μm full-width at half-maximum in diameter with a pair of Kirkpatrick-Baez mirrors. The studied crystal inside the DAC was aligned to the rotation centre of the diffractometer. An X-ray sensitive charge-coupled device was positioned at the desired diffraction angle, 1 m from the sample. The off-specular (111) reflection of the gold crystal was chosen to allow separation of the signals from multiple crystals in the beam. To follow the same particle after changing pressure, a local search in reciprocal space was performed to pick an isolated single crystal within half a degree along the 2 theta arc to guarantee only one (111) reflection in this region. Once the particular grain was chosen, we also checked the sample stage in the plane perpendicular to the incident beam to ensure no similar oriented crystals were found within three times the beamsize (~5 microns). To measure its full 3D diffraction patterns, the crystal was rotated by 0.4 degree with 0.01 degree step size. At each rotation angle, a two-dimensional frame of the 3D far-field diffraction pattern was recorded by the charge-coupled device. By stacking all these two-dimensional diffraction frames together, a complete 3D diffraction pattern was obtained, from which real-space images can be reconstructed, solving the phase problem by oversampling and a support constraint [11] . An online ruby system was installed above the DAC to monitor the pressure in situ , which allows one to change pressure without taking the cell off the sample stage. How to cite this article: Yang, W. et al . Coherent diffraction imaging of nanoscale strain evolution in a single crystal under high pressure. Nat. Commun. 4:1680 doi: 10.1038/ncomms2661 (2013).